The antiparasitic drug ivermectin is a novel FXR ligand that regulates metabolism Farnesoid X receptor (FXR) has important roles in maintaining bile acid and cholesterol homeostasis. Here we report that the antiparasitic drug ivermectin is a ligand for nuclear FXR. We identify ivermectin using a high-throughput compound library screening and show that it induces the transcriptional activity of the FXR with distinctive properties in modulating coregulator recruitment. The crystal structure of ivermectin complexed with the ligand-binding domain of FXR reveals a unique binding mode of ivermectin in the FXR ligand-binding pocket, including the highly dynamic AF-2 helix and an expanded ligand-binding pocket. Treatment of wild-type mice, but not of FXR-null mice, with ivermectin decreases serum glucose and cholesterol levels, suggesting that ivermectin regulates metabolism through FXR. Our results establish FXR as the first mammalian protein targeted by ivermectin with high selectivity. Considering that ivermectin is a widely used clinical drug, our findings reveal a safe template for the design of novel FXR ligands. Ivermectin (Stromectol or Ivomec) is a macrocyclic lactone derived from avermectin, which is produced by an actinomycete, Streptomyces avermitilis [1] . As a clinical drug against a variety of nematode and arthropod parasites through the mediation of neurotransmission, ivermectin is widely used for the treatment and control of human filarial infections and parasites in livestock [2] . It is highly effective and safe, and is well tolerated with a single annual oral dose in human. The binding of ivermectin to γ-aminobutyric acid receptors increases the releasing of inhibitory neurotransmitter γ-aminobutyric acid in parasite, resulting in the blocking of the transmission of nerve signals, which leads to nerve palsy, loss of contractility of the muscle cells and, ultimately, parasite death [3] , [4] , [5] , [6] . Recently, Hibbs et al . [7] provided the first intuitive evidence for ivermectin to act in parasite by solving the crystal structure of the glutamate-gated Cl − channel receptor binding to ivermectin. As a drug targeting nematode and arthropod parasites, ivermectin has not been reported to directly interact with any mammalian proteins with high selectivity. Farnesoid X receptor (FXR), also known as bile acid receptor, is a member of the nuclear hormone receptor superfamily that is highly expressed in mammalian liver, intestine, kidney and adrenal gland [8] , [9] , [10] . Following the ligand binding, the transcriptional function of FXR is mediated through the recruitment or release of specific coregulators, including coactivators such as SRC1 and corepressors such as NCoR and SMRT [11] , [12] , [13] . FXR has important roles in maintaining bile acid and cholesterol homeostasis by regulating genes, such as cholesterol 7α-hydroxylase ( CYP7A1 ) [14] , [15] , [16] . In recent years, increasing evidence showed that activation of FXR by agonists, such as bile acids and GW4064, also had critical roles in regulating glucose homeostasis and insulin sensitivity [17] , [18] , [19] , [20] , [21] , [22] . Activation of FXR by agonists or hepatic overexpression of constitutively active FXR lowered blood glucose levels in both diabetic db/db and high-fat diet-fed wild-type mice by downregulating the critical enzymes involved in gluconeogenesis, such as phosphoenolpyruvate carboxykinase (PEPCK) and glucose 6-phosphatase (G6Pase) . Consistently, FXR-null mice exhibited glucose intolerance and insulin insensitivity [22] . Despite the considerable attention of FXR as a key regulator in metabolism, the therapeutic potentials of FXR ligands remain to be further studied [16] , [23] . As a natural FXR ligand, bile acid chenodeoxycholic acid (CDCA) binds to FXR with only micromolar affinity, and has potential risks of cell toxicity at concentrations above 100 μM (ref. 13 ). Further, bile acids also activate other nuclear receptor, such as VDR and pregnane X receptor (PXR), as well as TGR5 membrane receptor [13] . As such, CDCA is an FXR ligand with poor selectivity and low affinity. Many synthetic FXR ligands have also been described, but have limitations owing to side effects and uncertain bioavailability. For example, GW4064, the most widely used synthetic FXR ligand, shows ambiguous results in regulating glucose homeostasis [16] . Therefore, a new drug-design strategy will be of great use for developing novel FXR ligands with therapeutic potentials in treating metabolic syndrome. In this study we report the identification of nuclear receptor FXR as a novel target for ivermectin, an antiparasitic drug. Both the transactivation and binding assays suggest that ivermectin is a highly selective FXR ligand with unique properties in modulating coregulator recruitment. The structure of FXR complexed with ivermectin shows a unique binding mode of ivermectin in the FXR ligand-binding pocket. Remarkably, ivermectin displays antidiabetic activities by reducing blood glucose and cholesterol levels, and also by improving insulin sensitivity in an FXR-dependent manner. Our observations therefore indicate that ivermectin may represent a unique safe approach for designing novel FXR ligands for the therapeutic purpose. Identification of ivermectin as a novel FXR ligand To identify new FXR agonists from the safe drugs on the market, we screened Biomol FDA (Food and Drug Administration) chemical libraries based on AlphaScreen biochemical assay, which is widely used for detecting ligand-dependent interaction between nuclear receptors and their coactivators [24] , [25] . To our surprise, ivermectin, a widely used antiparasitic drug with a chemical structure distinct from FXR ligands GW4064 and CDCA, strongly promoted the coactivator recruitment by FXR ( Supplementary Fig. S1 ). As shown in Fig. 1a , ivermectin enhanced the interaction of FXR with various coactivator LXXLL motifs from the family of steroid receptor coactivators (SRC1-2, SRC2-3 and SRC3-3), with a less extent than that of GW4064 ( Fig. 1a ). Notably, ivermectin also induced the recruitment of corepressor NCoR-2 by FXR, which is distinct from GW4064 ( Fig. 1a ). The ability of ivermectin to induce the recruitment of corepressor NCoR-2 by FXR was further validated by mammalian two-hybrid assays ( Supplementary Fig. S2 ). We also performed peptide-profiling experiments using a panel of 16 unlabelled peptides ( Supplementary Table S3 ) selected from both coactivators and corepressors to compete off the binding of the second LXXLL motif of SRC1 (SRC1-2) to FXR in response to ivermectin binding ( Supplementary Fig. S3 ). Consistent with the results above, corepressor motifs, including SMRT-2 and NCoR-2, substantially inhibited the SRC1 binding to ivermectin-bound FXR but not GW4064-bound FXR, whereas most coactivator LXXLL motifs have similar peptide profiles for both ligands. Our results suggest a partial agonist nature of ivermectin with unique properties in modulating coregulator recruitment. 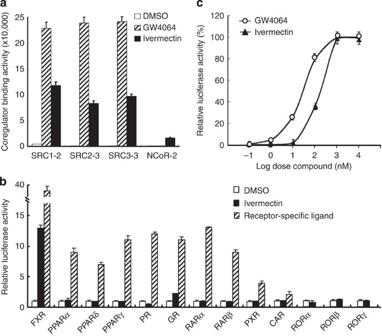Figure 1: Identification of ivermectin as a novel FXR ligand. (a) Various coregulator binding motifs bind to FXR in response to 0.5 μM ivermectin or GW4064 by AlphaScreen assay. The peptide sequences are listed in Methods. (b) Receptor-specific transactivation by ivermectin. COS-7 cells were cotransfected with plasmids encoding full-length nuclear receptors and their cognate response reporters, respectively (seeMethods). After transfection, cells were treated with dimethyl sulphoxide (DMSO), 0.5 μM ivermectin or ligands specific for each receptor: FXR, 0.5 μM GW4064; peroxisome proliferator-activated receptor (PPAR)α, 1 μM GW590735; PPARδ, 1 μM GW0472; PPARγ, 1 μM rosiglitazone; GR, 0.1 μM dexamethasone; progesterone receptor (PR), 0.1 μM progesterone; RARα and RARβ, 1 μM all-trans-retinoic acid; PXR, 10 μM rifampicin; constitutive androstane receptor (CAR), 5 μM CITCO. (c) Dose responses of ivermectin in transactivating FXR. COS-7 cells were cotransfected with full-length FXRα and an EcRE luciferase reporter. After transfection for 5 h, cells were treated with various concentrations of ivermectin or GW4064. Forbandc, luciferase data were normalized to renilla activity cotransfected as an internal control. Values are the means±s.e.m. of three independent experiments. Figure 1: Identification of ivermectin as a novel FXR ligand. ( a ) Various coregulator binding motifs bind to FXR in response to 0.5 μM ivermectin or GW4064 by AlphaScreen assay. The peptide sequences are listed in Methods. ( b ) Receptor-specific transactivation by ivermectin. COS-7 cells were cotransfected with plasmids encoding full-length nuclear receptors and their cognate response reporters, respectively (see Methods ). After transfection, cells were treated with dimethyl sulphoxide (DMSO), 0.5 μM ivermectin or ligands specific for each receptor: FXR, 0.5 μM GW4064; peroxisome proliferator-activated receptor (PPAR)α, 1 μM GW590735; PPARδ, 1 μM GW0472; PPARγ, 1 μM rosiglitazone; GR, 0.1 μM dexamethasone; progesterone receptor (PR), 0.1 μM progesterone; RARα and RARβ, 1 μM all-trans-retinoic acid; PXR, 10 μM rifampicin; constitutive androstane receptor (CAR), 5 μM CITCO. ( c ) Dose responses of ivermectin in transactivating FXR. COS-7 cells were cotransfected with full-length FXRα and an EcRE luciferase reporter. After transfection for 5 h, cells were treated with various concentrations of ivermectin or GW4064. For b and c , luciferase data were normalized to renilla activity cotransfected as an internal control. Values are the means±s.e.m. of three independent experiments. Full size image To probe the physiological roles of ivermectin in FXR signalling, cell-based reporter assay was employed to characterize the transcriptional properties of FXR in response to ivermectin. COS-7 cells were cotransfected with plasmids encoding full-length FXRα and other nuclear receptors, respectively, together with their cognate response reporters. In agreement with initial library screen results, ivermectin significantly transactivated FXR using an EcRE reporter, with a weaker activity than GW4064, but had no substantial impact on other nuclear receptors tested, including peroxisome proliferator-activated receptor-α, -δ and -γ, progesterone receptor, PXR, constitutive androstane receptor, retinoic acid receptor (RAR) -α and -β, and retinoic acid-related receptor-α, -β and -γ ( Fig. 1b ). The FXR-specific transactivation by ivermectin was further validated by mammalian two-hybrid assays ( Supplementary Fig. S4 ). Of note, ivermectin had a minimal effect on glucocorticoid receptor (GR) full length but not GR ligand-binding domain (LBD) ( Fig. 1b and Supplementary Fig. S4 ). Furthermore, full-dose curves revealed that ivermectin activated FXR in a concentration-dependent manner with an EC50 of ~200 nM ( Fig. 1c ), suggesting that ivermectin is a highly potent FXR ligand. The functional properties of ivermectin to activate FXR with four different FXR response elements [26] , in addition to EcRE, were also analysed and similar results were obtained ( Supplementary Fig. S5 ). Structure of the FXR LBD in complex with ivermectin To determine the molecular basis for the recognition of FXR by ivermectin, we solved the crystal structure of FXR LBD complexed with ivermectin. The data statistics and the refined structures are summarized in Supplementary Table S1 . The structure reveals that the ivermectin-bound FXR LBD adopts a three-layer helical sandwich arrangement that resembles most nuclear receptor structures ( Fig. 2a ) [27] , [28] . Notably, carboxy terminal AF-2 helix is invisible due to very low and ambiguous electron density, suggesting a highly flexible and dynamic nature of AF-2 helix induced by ivermectin binding ( Fig. 2a and Fig. 3a ), which is consistent with its relatively weaker induction on FXR transcriptional activity and coactivator recruitment compared with GW4064. Inside the ligand-binding pocket of FXR, the existence of ivermectin was apparent from the highly revealing electron density map shown in Fig. 2b . Superposition of structures of FXR/ivermectin and FXR/GW4064 (ref. 29 ) revealed that both ligand-bound FXR LBDs aligned well with ligands occupying the similar binding site in the FXR pocket ( Fig. 3 ). However, both helix 2 and helix 6 were shifted outward and also distorted to make extra space to accommodate the larger size of ivermectin, resulting in the substantial expansion of the pocket size in comparison with GW4064-bound FXR LBD ( Fig. 3c ). The conformational changes of FXR pocket induced by ivermectin indicate that FXR has a great flexibility to adapt to the binding of diverse ligands. 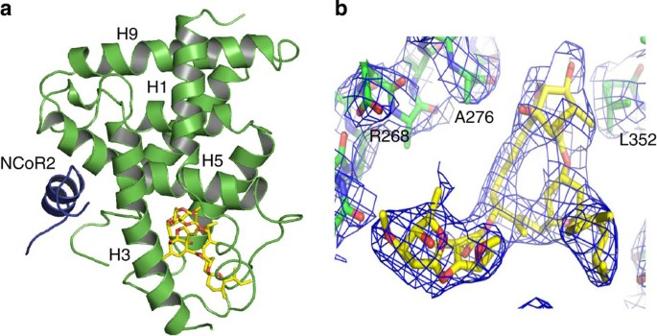Figure 2: Structural determination of the FXR LBD in complex with ivermectin. (a) The structure of ivermectin bound with FXR LBD in ribbon representation. FXR LBD is coloured in green and the NCoR-2 motif is in blue. The bound ivermectin is shown in stick representation with carbon and oxygen atoms depicted in yellow and red, respectively. (b) 2Fo-Fc electron density map (1.0σ) showing the bound ivermectin to the FXR LBD. Figure 2: Structural determination of the FXR LBD in complex with ivermectin. ( a ) The structure of ivermectin bound with FXR LBD in ribbon representation. FXR LBD is coloured in green and the NCoR-2 motif is in blue. The bound ivermectin is shown in stick representation with carbon and oxygen atoms depicted in yellow and red, respectively. ( b ) 2Fo-Fc electron density map (1.0σ) showing the bound ivermectin to the FXR LBD. 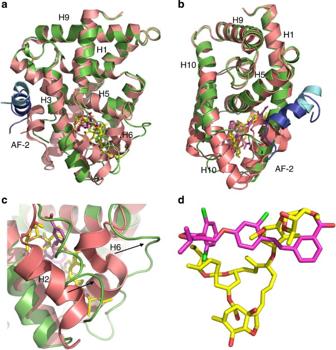Figure 3: Conformational changes of FXR LBD induced by ivermectin binding. (a–c) Superposition of the FXR–ivermectin structure (FXR is in green and NCoR-2 motif is in blue ) with the FXR–GW4064 structure (FXR is in salmon red and the SRC1 peptide is in cyan), showing the destabilization of helix12 (a,b) and the pocket size expansion (c) characterized by the conformational changes of helix 2 and helix 6 induced by the binding of ivermectin (indicated by arrows). Ivermectin is in yellow and GW4064 is in purple. (d) Superposition of ivermectin (yellow) with GW4064 (purple). Full size image Figure 3: Conformational changes of FXR LBD induced by ivermectin binding. ( a – c ) Superposition of the FXR–ivermectin structure (FXR is in green and NCoR-2 motif is in blue ) with the FXR–GW4064 structure (FXR is in salmon red and the SRC1 peptide is in cyan), showing the destabilization of helix12 ( a , b ) and the pocket size expansion ( c ) characterized by the conformational changes of helix 2 and helix 6 induced by the binding of ivermectin (indicated by arrows). Ivermectin is in yellow and GW4064 is in purple. ( d ) Superposition of ivermectin (yellow) with GW4064 (purple). Full size image Functional correlation of the ivermectin–FXR interaction To validate the roles of pocket residues in ivermectin binding and FXR activation, we mutated several key residues that contact different groups of ivermectin and tested the transcriptional activity of these mutated FXR in response to ivermectin in cell-based reporter assays using full-length FXR and the EcRE reporter. A291W mutation was designed to reduce the size of the FXR pocket by changing the corresponding residue to a tryptophan ( Fig. 4 and Supplementary Fig. S6A ), thereby preventing the binding of the bulky FXR ligands. As expected, this mutation abolished the FXR transcriptional activity by both GW4064 and ivermectin ( Fig. 4e . The hydrophobic side chain of F284 stabilizes the ligand binding by making hydrophobic interactions with both GW4064 and ivermectin. Despite the loss of hydrophobic contacts with both ligands, F284H mutation was predicted to initiate hydrogen bonds with a nitrogen atom on GW4064 but not ivermectin ( Fig. 4b and Supplementary Fig. S6B ). Accordingly, this mutant abolished ivermectin-mediated FXR transcriptional activity but retained the ability to be activated by GW4064 ( Fig. 4e ). Consistent with Fig. 4e , AlphaScreen assays showed that the F284H mutant substantially disrupted the binding of the NCoR-2 peptide and also the SRC1-2 peptide in response to ivermectin ( Supplementary Fig. S6E ), further affirming that the FXR ligand-binding pocket has unique properties that dictate the discrimination between ivermectin and GW4064. In contrast, mutations on L287 and H447 ( Fig. 4c and Supplementary Fig. S6C,D ) abolished or substantially reduced GW4064-mediated FXR transcriptional activity, but they increased the ability to be activated by ivermectin ( Fig. 4e ). Taken together, our mutagenic analyses showed distinct results on the activation of FXR by ivermectin and GW4064, highlighting the differential roles of FXR pocket residues in recognizing various ligands. 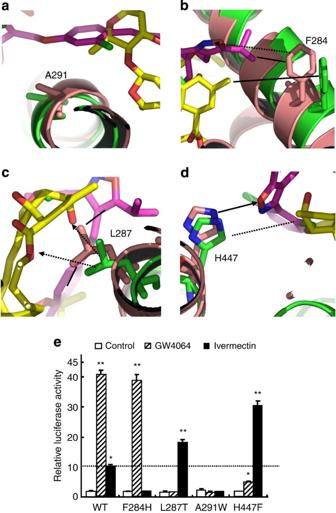Figure 4: Functional correlation of the ivermectin/FXR interactions. (a–d) Molecular determinants of the interaction between FXR with ligand ivermectin. Overlays of the FXR–ivermectin structure (green) with the FXR–GW4064 (salmon red) structure, where ligand ivermectin is in yellow and GW4064 is in purple. The hydrophobic interactions and hydrogen bonds are shown with lines and arrows, respectively. The potential hydrophobic interactions and hydrogen bonds, if the corresponding mutations are made as indicated in e, are shown in dashed lines and dashed arrows, respectively. (e) Differential effects of mutations of key FXR residues on its transcriptional activity in response to ivermectin and GW4064 in cell-based reporter assays. COS-7 cells were cotransfected with plasmids encoding full-length wild-type (WT) FXR or FXR mutants as indicated in the figure, together with an EcRE luciferase reporter. The cells were treated with 0.5 μM ivermectin and GW4064, respectively. The dashed line indicates the activation level of WT FXR by ivermectin. Values are the means±s.e.m. of three independent experiments. *P<0.05, **P<0.01 versus vehicle, Student’st-test. Figure 4: Functional correlation of the ivermectin/FXR interactions. ( a – d ) Molecular determinants of the interaction between FXR with ligand ivermectin. Overlays of the FXR–ivermectin structure (green) with the FXR–GW4064 (salmon red) structure, where ligand ivermectin is in yellow and GW4064 is in purple. The hydrophobic interactions and hydrogen bonds are shown with lines and arrows, respectively. The potential hydrophobic interactions and hydrogen bonds, if the corresponding mutations are made as indicated in e, are shown in dashed lines and dashed arrows, respectively. ( e ) Differential effects of mutations of key FXR residues on its transcriptional activity in response to ivermectin and GW4064 in cell-based reporter assays. COS-7 cells were cotransfected with plasmids encoding full-length wild-type (WT) FXR or FXR mutants as indicated in the figure, together with an EcRE luciferase reporter. The cells were treated with 0.5 μM ivermectin and GW4064, respectively. The dashed line indicates the activation level of WT FXR by ivermectin. Values are the means±s.e.m. of three independent experiments. * P <0.05, ** P <0.01 versus vehicle, Student’s t -test. Full size image Metabolic effects of ivermectin in mice on a high-fat diet To investigate whether ivermectin has effects on glucose and cholesterol metabolism in vivo as a FXR ligand, wild-type and FXR –/– mice were fed with high-fat diet and intraperitoneally (i.p.) injected daily with vehicle or ivermectin for 14 days. Of note, no liver injury of ivermectin treatment was observed when evaluated by aspartate aminotransferase, alanine aminotransferase and liver histology ( Supplementary Fig. S7 ), in consistency with published results [30] , [31] . Interestingly, serum glucose and cholesterol, including high-density lipoprotein and low-density lipoprotein (LDL)/very LDL levels, were significantly decreased in wild-type mice after treatment with ivermectin ( Fig. 5 and Supplementary Fig. S8 ), whereas ivermectin treatment had no effect on food intake and body weight ( Fig. 5a ). In contrast, no significant differences of serum glucose and cholesterol levels were observed by ivermectin treatment in FXR –/– mice. Notably, the serum insulin level was significantly decreased in ivermectin-treated wild-type mice ( Fig. 5d ), suggesting that ivermectin might have lowered the serum glucose levels through improving insulin sensitivity. Indeed, ivermectin-injected mice showed improved insulin sensitivity as well as glucose tolerance compared with vehicle-treated controls ( Supplementary Fig. S9 ). We conclude that ivermectin is capable of regulating serum glucose and cholesterol levels by directly targeting FXR. 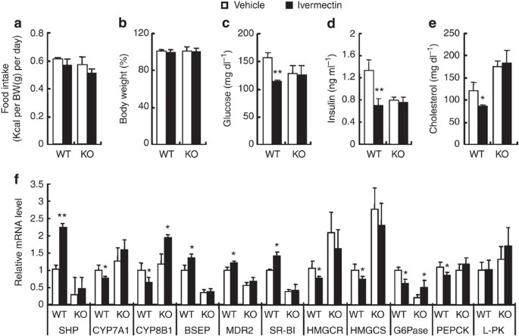Figure 5: Ivermectin regulates metabolic parameters in a FXR-dependent manner. Wild-type (WT) and FXR−/−(knock-out (KO)) mice were fed with high-fat diet and i.p. injected with vehicle or ivermectin (1.3 mg kg−1) once a day for 14 days (n=6 per group for all data in this figure). The food intake were measured every second day. (a) Food intake. Kcal, kilocalories; BW, body weight. After 6 h of fasting, mice were weighed and the body weights were indicated as percentage (%) of the initial weight of mice (b). Serum was collected and the levels of serum glucose (c), insulin (d) and cholesterol (e) were determined. (f) Hepatic mRNA levels of metabolism-related genes were quantified by real-time PCR and normalized to actin. Values are the means±s.e.m. of six independent experiments. *P<0.05, **P<0.01 versus vehicle, Student’st-test. Figure 5: Ivermectin regulates metabolic parameters in a FXR-dependent manner. Wild-type (WT) and FXR −/− (knock-out (KO)) mice were fed with high-fat diet and i.p. injected with vehicle or ivermectin (1.3 mg kg −1 ) once a day for 14 days ( n =6 per group for all data in this figure). The food intake were measured every second day. ( a ) Food intake. Kcal, kilocalories; BW, body weight. After 6 h of fasting, mice were weighed and the body weights were indicated as percentage (%) of the initial weight of mice ( b ). Serum was collected and the levels of serum glucose ( c ), insulin ( d ) and cholesterol ( e ) were determined. ( f ) Hepatic mRNA levels of metabolism-related genes were quantified by real-time PCR and normalized to actin. Values are the means±s.e.m. of six independent experiments. * P <0.05, ** P <0.01 versus vehicle, Student’s t -test. Full size image To further assess the molecular mechanisms underlying the physiological functions of ivermectin, we measured the mRNA levels of metabolism-related genes in liver tissues of mice treated with either vehicle or ivermectin ( Fig. 5f ). Data from quantitative PCR revealed that ivermectin treatment induced hepatic mRNA levels of SHP, while it reduced the mRNA levels of CYP7A1 and CYP8B1, three well-characterized FXR direct or indirect target genes, in wild-type but not FXR –/– mice, reaffirming that ivermectin is an FXR ligand in vivo . Consistent with the metabolic benefits of ivermectin, the expression of PEPCK and G6Pase, two critical enzymes involved in gluconeogenesis, was significantly reduced in ivermectin-treated wild-type mice, but not in FXR –/– mice ( Fig. 5f ), also in agreement with the previous reports that FXR agonist cholic acid suppressed PEPCK and G6Pase gene expression through FXR (ref. 21 ). In contrast to GW4064, ivermectin showed no significant inhibition of L-PK mRNA levels in both primary hepatocytes and liver tissues ( Fig. 6f and Supplementary Fig. S10 ), the regulation associated with the ambiguous effects of GW4064 on glucose metabolism [16] , [32] . Genes associated with cholesterol metabolism were also regulated by ivermectin treatment ( Fig. 5f ). The mRNA levels of the class B, type-I scavenger receptor, the bile salt excretory pump and the multidrug resistance gene 2 were all induced in the liver tissues in ivermectin-treated wild-type but not FXR −/− mice ( Fig. 5f ). Meanwhile, the rate-limiting enzymes of cholesterol biosynthesis, hydroxymethylglutaryl coenzyme A synthase and hydroxymethylglutaryl coenzyme A reductase [33] , [34] , were significantly downregulated by ivermectin, also in an FXR-dependent manner ( Fig. 5f ). These results reaffirm that ivermectin regulates gene expression, and glucose and cholesterol homeostasis in an FXR-dependent manner. 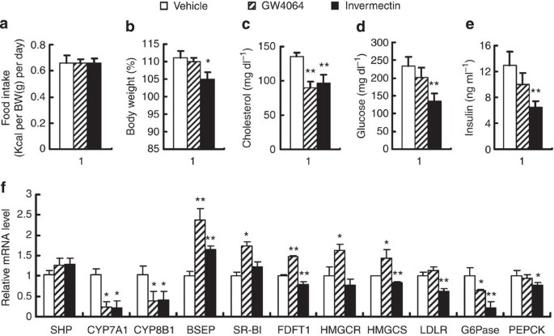Figure 6: Ivermectin treatment improves hyperglycemia and hyperlipidemia in diabetic KK-Ay mice. KK-Ay mice were fed with high-fat diet and i.p. injected with vehicle, ivermectin (1.3 mg kg−1) or GW4064 (30 mg kg−1) once a day for 14 days (n=6 per group for all data in this figure). The food intake were measured every second day. (a) Food intake. Kcal, kilocalories; BW, body weight. After 6 h of fasting, mice were weighed and the body weights were indicated as percentage (%) of the initial weight of mice (b). Serum was collected and serum cholesterol (c), glucose (d) and insulin (e) levels were determined. (f) Hepatic mRNA levels of metabolism-related genes were quantified by real-time PCR and normalized to actin. Values are the means±s.e.m. of six independent experiments. *P<0.05, **P<0.01 versus vehicle, Student’st-test. Figure 6: Ivermectin treatment improves hyperglycemia and hyperlipidemia in diabetic KK-Ay mice. KK-Ay mice were fed with high-fat diet and i.p. injected with vehicle, ivermectin (1.3 mg kg −1 ) or GW4064 (30 mg kg −1 ) once a day for 14 days ( n =6 per group for all data in this figure). The food intake were measured every second day. ( a ) Food intake. Kcal, kilocalories; BW, body weight. After 6 h of fasting, mice were weighed and the body weights were indicated as percentage (%) of the initial weight of mice ( b ). Serum was collected and serum cholesterol ( c ), glucose ( d ) and insulin ( e ) levels were determined. ( f ) Hepatic mRNA levels of metabolism-related genes were quantified by real-time PCR and normalized to actin. Values are the means±s.e.m. of six independent experiments. * P <0.05, ** P <0.01 versus vehicle, Student’s t -test. Full size image Metabolic effects of ivermectin in diabetic KK-Ay mice To further study whether ivermectin treatment improves hyperglycemia and hyperlipidemia in a diabetic mouse model as an FXR ligand, KK-Ay mice were fed with high-fat diet and i.p. injected daily with vehicle, GW4064 or ivermectin. GW4064 and ivermectin treatment had no effect on food intake ( Fig. 6a ), whereas ivermectin treatment reduced KK-Ay body weight compared with vehicle and GW4064 treatment ( Fig. 6b ). Both GW4064 and ivermectin significantly lowered serum cholesterol levels ( Fig.6c ). Consistent with the results on wild-type mice, ivermectin treatment displayed similar metabolic impact on serum glucose and insulin levels in diabetic KK-Ay mice ( Figs. 6d ). In contrast, GW4064 showed little effect. To assess whether gene expression in KK-Ay mice were affected by ivermectin treatment, we analysed genes related with glucose and cholesterol metabolism ( Fig. 6f ). As expected, CYP7A1 and CYP8B1 were reduced by GW4064 and ivermectin treatment. Furthermore, ivermectin treatment elicited either no induction or significant suppression of the mRNA levels of genes involved in cholesterol synthesis, such as FDFT1 (farnesyl-diphosphate farnesyltransferase 1), hydroxymethylglutaryl coenzyme A synthase, LDL receptor and hydroxymethylglutaryl coenzyme A reductase ( Fig. 6f ), which is also in contrast to the results from GW4064. In addition, ivermectin also showed more favourable regulations on G6Pase and PEPCK than on GW4064 ( Fig. 6f ). Together, these results demonstrated that ivermectin can effectively improve hyperglycemia and hyperlipidemia in diabetes model mice by regulating genes expression, with potential advantages over GW4064 in improving hyperglycemia and hypercholesterolemia as an FXR ligand. The nuclear receptors are important drug targets due to their regulation functions in physiological and also pathological processes. Given the important roles of FXR in a variety of physiological and pathological processes, the ligands that regulate FXR activity are promising therapeutic agents for different diseases. Compared with many other nuclear receptors, the clinical applications of FXR ligands remain much less developed. We describe here the identification and characterization of ivermectin as a unique FXR ligand ( Fig. 1 ). Ivermectin binds in the pocket of FXR with a distinctive binding mode owing to its distinct molecular size and structure compared with other ligands ( Fig. 2 , and Figs 3 and 4 ), such as GW4064 (ref. 29 ), fexaramine [35] and CDCA [36] , which provides another evidence for the conformational flexibility of nuclear receptors to adapt diverse ligands. More importantly, ivermectin treatment can downregulate serum glucose and cholesterol levels by directly targeting FXR ( Figs 5 and 6 ). Previous reports also showed that activation of FXR by the synthetic agonist GW4064 or hepatic overexpression of constitutively active FXR significantly lowered serum glucose levels in both wild-type mice and diabetic mice models (db/db and KK-Ay mice) in an FXR-dependent manner by regulating related genes [21] , [22] . However, recent observations of glucose level regulation by FXR agonist GW4064 remains ambiguous, as some reports suggested that activation of FXR with GW4064 in wild-type or diabetic mice did not improve hyperglycemia [17] , [37] . Although the gluconeogenesis gene G6Pase was reduced with GW4064 treatment in our studies, no effects on serum glucose and insulin levels were observed. However, our studies demonstrated much more favourable effects of ivermectin on glucose and insulin homeostasis in both wild-type and KK-Ay mice by regulating related genes. Further, our results showed that ivermectin treatment had no obvious body weight gain, which is a side effect of GW4064 (ref. 38 ). Together, our results suggest that ivermectin as a novel FXR ligand may possess advantages over GW4064 in regulating glucose homeostasis. The distinctive functional profile of nuclear receptors in response of various ligand binding is largely determined by the selective usage of transcriptional coregulators, as ligand-specific recruitment of coregulators ultimately controls transcriptional output of direct and indirect target genes. Thus, ligand-bound FXR may show diverse pharmacological functions depending on the specific binding of coregulators induced by different ligands. The results from both biochemical AlphaScreen assay and cell-based reporter assay showed that ivermectin is a partial agonist for FXR owing to its much less capability in recruiting coactivators compared with typical full agonist GW4064 ( Fig. 1 ). Unlike a typical full agonist, such as GW4064, ivermectin-bound FXR has a marked binding preference for the corepressor motifs, including SMRT-2 and NCoR-2 ( Fig. 1a and Supplementary Fig. S2 ). Consistent with these results, the crystal structure of the ivermectin/FXR complex reveals a highly dynamic AF-2 helix, which is critical for nuclear receptors to interact with coregulators ( Fig. 3 ). Thus, the selective usage of coregulators may contribute to the unique characteristics of ivermectin in modulating FXR activity in metabolism. Considering that ivermectin is already a clinical drug approved by the FDA, our findings reveal an alternative template for design of FXR ligands with therapeutic potentials to rapid clinical applications by providing a safe lead compound. Moreover, given the fact that the molecular targets of many FDA drugs are still not clear [39] , our study also validates a powerful screening strategy for the search of novel lead compounds for nuclear receptors as well as other molecular targets based on existing drugs, which also opens up many potentials for old drugs. Protein preparation The human FXR LBD (residues 243–472) was expressed as an amino-terminal 6 × His fusion protein from the expression vector pET24a (Novagen). BL21 (DE3) cells transformed with expression plasmids were grown in lysogeny broth at 25 °C to an OD600 of ~1.0 and induced with 0.1 mM isopropyl 1-thio-β- D -galactopyranoside at 16 °C. Cells were collected and sonicated in 200 ml extraction buffer (20 mM Tris pH 8.0, 150 mM NaCl, 10% glycerol and 25 mM imidazole) per 6 l of cells. The lysate was centrifuged at 20,000 r.p.m. for 30 min and the supernatant was loaded on a 5-ml NiSO 4 -loaded HiTrap HP column (GE Healthcare). The column was washed with extraction buffer and the protein was eluted with a gradient of 25–500 mM imidazole. The FXR LBD was further purified with a Q-Sepharose column (Amersham Biosciences). To prepare the protein–ligand complex, we added a fivefold molar excess of the ivermectin to the purified protein, followed by filter concentration to 10 mg ml −1 . The FXR LBD was complexed with a twofold molar of a NCoR peptide (PASNLGLEDIIRKALMGS) before filter concentration. Cofactor binding assays The binding of the various peptide motifs to FXR LBD in response to ligands was determined by AlphaScreen assays using a hexahistidine detection kit from Perkins-Elmer as described before [25] . The experiments were conducted with ~20–40 nM receptor LBD and 20 nM biotinylated cofactor peptides in the presence of 5 μg ml −1 donor and acceptor beads in a buffer containing 50 mM MOPS, 50 mM NaF, 0.05 mM CHAPS and 0.1 mg ml −1 BSA, all adjusted to pH 7.4. The peptides with an N-terminal biotinylation are listed below. SRC1-2, SPSSHSSLTERHKILHRLLQEGSP; SRC2-3, QEPVSPKKKENALLRYLLDKDDTKD; SRC3-3, PDAASKHKQLSELLRGGSG; NCoR-2, GHSFADPASNLGLEDIIRKALMGSF. Crystallization and structure determination The crystals of FXR/ivermectin complex were grown at room temperature in hanging drops containing 1.0 μl of the above ligand–protein solutions and 1.0 μl of well buffer containing 50 mM HEPES pH 7.0 and 3.5 M sodium formate. The crystals were directly flash-frozen in liquid nitrogen for data collection. The observed reflections were reduced, merged and scaled with DENZO and SCALEPACK in the HKL2000 package [40] . The structures were determined by molecular replacement in the CCP4 suite. Manual model building was carried out with Coot [41] followed by REFMAC refinement in the CCP4 suite. Transient transfection assay COS-7 cells were maintained in DMEM containing 10% fetal bovine serum and were transiently transfected using Lipofectamine 2000 (Invitrogen) [42] . All mutant FXR plasmids were created using the Quick-Change site-directed mutagenesis kit (Stratagene). Before 24 h of transfection, 24-well plates were plated (5 × 10 4 cells per well). The cells were cotransfected with plasmids encoding full-length nuclear receptors and their cognate luciferase reporters as follows: human FXRα with EcRE-Luc, human peroxisome proliferator-activated receptors (α, δ and γ) with PPRE-Luc; human retinoic acid-related receptors (α, β and γ) with the Pcp2/RORE-Luc; human GR or progesterone receptor with the MMTV-Luc; human RARα or RARβ with βRE-Luc reporter; and human PXR and constitutive androstane receptor with PBRE-luc reporter. Among these reporters, MMTV-luc contains one copy of the response elements and the others have three copies. Ligands were added 5 h after transfection. Cells were collected 24 h later for the luciferase assays. Luciferase activities were normalized to renilla activity cotransfected as an internal control. Animals and diets, or compounds C57BL/6J, homozygous FXR-deficient (FXR –/– ) mice [19] and KK-Ay mice were maintained under environmentally controlled conditions with free access to standard chow diet and water. Animal experiments were conducted in the barrier facility of the Laboratory Animal Center, Xiamen University, approved by the Institutional Animal Use and Care Committee of Xiamen University, China. Mice of 10–12 weeks of age were fed with high-fat diet containing 60% fat, 20% protein and 20% carbohydrate (Research Diets, D12492) and i.p. injected with either vehicle (40% of 2-hydroxypropyl-β-cyclodextrin, Sigma), or vehicle containing GW4064 (30 mg kg −1 , Sigma) or ivermectin (1.3 mg kg −1 ) once a day for 14 days. Mice were killed after 6 h of fasting, mice body were weighed, tissues were collected and frozen in liquid nitrogen for use, and serum were collected to measure metabolite parameters. Real-time PCR RNA was isolated using Tissue RNA kit (Omega Bio-Tek, GA). The first strand complementary DNA were obtained by TAKARA reverse transcription kit. Real-time quantitative PCR were performed on a CFX96 Real-Time PCR Detection System (Bio-Rad) using SYBR Premix Ex Taq (TAKARA). Relative mRNA expression levels were normalized to actin levels. The primers used in this assay were listed in the Supplementary Table S2 . Quantification of serum biomarkers Serum was drawn from compound-treated mice after 6 h fasting. Serum glucose and cholesterol were analysed using glucose oxidase method (Applygen, Beijing, China) and Cholesterol Assay Kit (Bioassay Systems, USA), respectively. Serum insulin levels were determined by enzyme-linked immunosorbent assay using ultra-sensitive mouse insulin kit (Crystal Chem. Inc., USA). Statistical analysis Results were expressed as mean±s.e.m. P -values were calculated by using Student’s t -test. Accession codes: Atomic coordinates and structure factors have been deposited in the Protein Data Bank under accession code 4II6 . How to cite this article: Jin, L. et al . The antiparasitic drug ivermectin is a novel FXR ligand that regulates metabolism. Nat. Commun. 4:1937 doi: 10.1038/ncomms2924 (2013).